High-resolution three-dimensional mapping of mRNA export through the nuclear pore The flow of genetic information is regulated by selective nucleocytoplasmic transport of messenger RNA:protein complexes (mRNPs) through the nuclear pore complexes (NPCs) of eukaryotic cells. However, the three-dimensional (3D) pathway taken by mRNPs as they transit through the NPC, and the kinetics and selectivity of transport, remain obscure. Here we employ single-molecule fluorescence microscopy with an unprecedented spatiotemporal accuracy of 8 nm and 2 ms to provide new insights into the mechanism of nuclear mRNP export in live human cells. We find that mRNPs exiting the nucleus are decelerated and selected at the centre of the NPC, and adopt a fast-slow-fast diffusion pattern during their brief, ~12 ms, interaction with the NPC. A 3D reconstruction of the export route indicates that mRNPs primarily interact with the periphery on the nucleoplasmic side and in the centre of the NPC, without entering the central axial conduit utilized for passive diffusion of small molecules, and eventually dissociate on the cytoplasmic side. In all eukaryotic cells, the flow of genetic information from DNA to mRNA to protein encounters a physical impediment, as the mRNA has to pass through the nuclear envelope (NE) [1] , [2] , [3] , [4] , [5] . The membrane-bound nuclear pore complex (NPC) acts as the major gateway that mediates selective nucleocytoplasmic transport of individual messenger RNA:protein complexes (mRNPs) [6] , [7] , [8] , although very large RNP complexes were recently reported to exit the nucleus through nuclear membrane budding [9] . As arguably the largest nanomachine of the cell with a length of ~200 nm and an inner diameter of ~50 nm (refs 10 , 11 , 12 , 13 ), the NPC consists of approximately 30 different nucleoporins (Nups), estimated at 8, 16 or 32 copies per NPC [14] , [15] , [16] , [17] , [18] . Over one-third of these Nups, natively unfolded and rich in phenylalanine–glycine (FG) repeats, form the selective gateway for nucleocytoplasmic transport [19] , [20] , [21] . Nuclear mRNA export through this gateway can be divided into assembly with protein cofactors to form an mRNP, trafficking through the NPC, and release into the cytoplasm for subsequent translation [1] , [2] . In human cells, the transport receptor protein Tap forms a heterodimer with cofactor p15 to facilitate mRNP export by interacting with the FG Nups [22] , [23] . After shuttling through the NPC, mRNPs are directionally dissociated into the cytoplasm by the essential mRNP export factors Gle1, IP6 and DDX at the location of Nup214 (refs 2 , 24 , 25 ). Electron microscopy has provided a high resolution, but static picture of some of the mRNP translocation steps [26] . Recently, the real-time imaging of dynamic nuclear export events of single mRNPs has become possible through super-registration wide-field epi-fluorescence and light-sheet fluorescence microscopy [6] , [7] , [8] . Despite this current level of understanding, however, most dynamic features of nuclear export remain obscure. We recently developed a single-molecule fluorescence imaging approach, termed single-point edge-excitation sub-diffraction (SPEED) microscopy, and used it to capture transient interactions between transiting molecules and the NPC in human cells that had escaped previous observation [20] , [27] , [28] , [29] . Combined with a deconvolution algorithm, SPEED microscopy further enabled us to distinguish the three-dimensional (3D) transport routes of passive and facilitated transport upon real-time trafficking through native intact NPCs, resulting in a refined nuclear transport mechanism [27] , [28] , [29] . Here we have expanded SPEED microscopy to measure the kinetics and map the 3D transport pathways of single mRNPs through NPCs in living cells, achieving a spatiotemporal accuracy of 8 nm and 2 ms. With an ~3-fold higher spatial and 10-fold higher temporal resolution than any previous measurements [6] , [7] , [8] and a 3D view of the mRNP transport route, critical details of the dynamic features and selectivity filter of nuclear mRNP export are finally coming into focus. 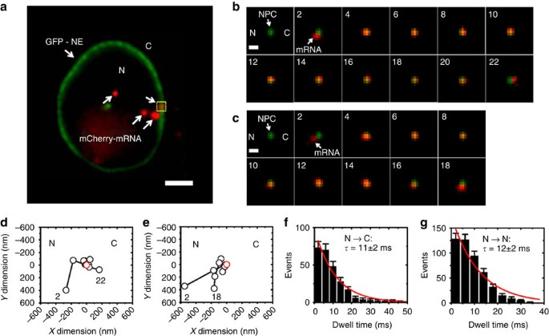Figure 1: Tracking single mRNPs through single NPCs. (a) Single mRNPs in the nucleus and on the NE imaged by wide-field epi-fluorescence. Four mCherry-tagged mRNP complexes (red spots) were observed, three in the nucleus and one on the GFP-NE (green rim). Scale bar, 5 μm. C, cytoplasm; N, nucleoplasm. (b) A typical successful single mRNP export event captured by SPEED microscopy. A single mCherry-tagged mRNP (red spot) started from the nucleus, interacted with a single GFP-tagged NPC (green spot) and arrived in the cytoplasm. Numbers denote time in milliseconds. (c) A typical abortive single mRNP export event. A single mCherry-tagged mRNP (red spot) started from nucleus, interacted with a single GFP-tagged NPC (green spot) and returned to the nucleus. (d,e) Single-particle tracks (black open dots) and the centroid of the NPC (red open dot) were acquired by 2D Gaussian fitting to point spread functions in a series of images for either the successful event inbor the abortive event inc. (f) Export time distribution of successful mRNP export events. Fitting with a mono-exponential decay function (red line) yielded the indicated export time. Error bars represent s.e.m. (g) Export time distribution of abortive mRNP export events. Error bars indicate s.e.m. SPEED microscopy of nuclear export of single mRNPs We conducted experiments in either HeLa cell lines expressing green fluorescent protein (GFP)-labelled NPCs and mCherry-tagged firefly luciferase mRNPs or in MEF cells with tdTomato-labelled NPCs and yellow fluorescent protein (YFP)-tagged β-actin mRNPs ( Table 1 , Methods). NPCs were labelled with typically eight copies of GFP or tdTomato ( Supplementary Fig. S1 ) and mRNPs with ~10 copies of tightly bound mCherry or YFP ( Supplementary Fig. S2 , Methods), and exported mRNPs showed typical diffusion properties in the cytoplasm ( Supplementary Fig. 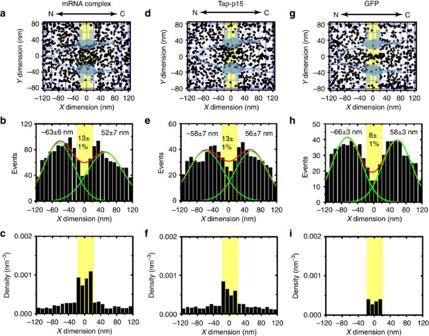Figure 2: 2D spatial distribution of molecular locations in the NPC. (a) Experimentally determined 2D spatial locations of mRNPs in the NPC. A schematic of the NPC (light blue) is superimposed, and the central region of the NPC (−20 nm to 20 nm) is highlighted in yellow. C, cytoplasmic side of the NPC; N, nucleoplasmic side of the NPC. (b) Gaussian fitting of the binned histogram of spatial mRNP locations along the NPC axis (xdimension) produced two major peaks on either side of the NPC. Approximately 13% of total localizations fall in the central channel of the NPC (−20 to 20 nm). (c) Density of spatial locations alongxdimension. (d–f) The 2D spatial locations, binned histogram of spatial locations along the NPC axis and corresponding spatial density for TapΔNLS–p15. (g–i) The 2D spatial locations, binned histogram of spatial locations along the NPC axis and corresponding spatial density for GFP. S3 and Table 2 ; we note that the dissociation of comparably dim single mCherry or YFP molecules from the multiply labelled mRNP remains invisible). Using SPEED microscopy ( Supplementary Figs S4 and S5 ), we illuminated a single labelled NPC in the NE and individual labelled mRNPs as they passed through this NPC (the average detection frequency is 0.6±0.2 mRNPs per pore per second obtained from 53 NPCs of 53 cells) with two different overlapped and focused laser beams, and the whole process was imaged using a CCD (charge-coupled device) camera at up to 500 frames per second ( Fig. 1a,b ). In each image sequence of an export event, the dynamic localizations of the mRNP relative to the centroid of NPC were tracked by Gaussian fitting ( Fig. 1b–e , Supplementary Movies 1 and 2 ), reaching 8–15 nm spatial resolution in living cells (Methods). Table 1 Dwell times and export efficiencies of mRNPs. Full size table Table 2 Diffusion coefficients of mRNPs. Full size table Figure 1: Tracking single mRNPs through single NPCs. ( a ) Single mRNPs in the nucleus and on the NE imaged by wide-field epi-fluorescence. Four mCherry-tagged mRNP complexes (red spots) were observed, three in the nucleus and one on the GFP-NE (green rim). Scale bar, 5 μm. C, cytoplasm; N, nucleoplasm. ( b ) A typical successful single mRNP export event captured by SPEED microscopy. A single mCherry-tagged mRNP (red spot) started from the nucleus, interacted with a single GFP-tagged NPC (green spot) and arrived in the cytoplasm. Numbers denote time in milliseconds. ( c ) A typical abortive single mRNP export event. A single mCherry-tagged mRNP (red spot) started from nucleus, interacted with a single GFP-tagged NPC (green spot) and returned to the nucleus. ( d , e ) Single-particle tracks (black open dots) and the centroid of the NPC (red open dot) were acquired by 2D Gaussian fitting to point spread functions in a series of images for either the successful event in b or the abortive event in c . ( f ) Export time distribution of successful mRNP export events. Fitting with a mono-exponential decay function (red line) yielded the indicated export time. Error bars represent s.e.m. ( g ) Export time distribution of abortive mRNP export events. Error bars indicate s.e.m. Full size image For firefly luciferase mRNPs, we found that 36±5% of all nuclear mRNP export events (total 201 events) were successful (that is, started from the nucleus, interacted with the NPC and arrived in the cytoplasm), whereas the remaining 64±5% events were aborted (that is, started from and returned to the nucleus after interacting with the NPC), consistent with previous reports [6] , [8] . The mRNP:NPC interaction times were similar at 11±2 ms (73 events) and 12±2 ms (128 events) for successful and abortive export events, respectively ( Fig. 1f,g ). To test the generality of our observations, the export efficiency and time for similar-sized, YFP-labelled β-actin mRNPs were measured under the same experimental conditions and were found to be the same as those for firefly luciferase mRNPs ( Table 1 ). Strikingly, the export times obtained for both mRNPs were more than 10-fold shorter than those previously reported for the same YFP-labelled β-actin mRNPs [6] , [7] . We found that this difference was at least in part related to the technical advances of SPEED microscopy, including: first, faster detection speed. Our detection time resolution of 2 ms per frame, 10 times faster than that previously achieved, enabled us to capture faster mRNA export events that may have escaped earlier observation. Indeed, when we lowered the detection resolution to 20 ms per frame, we found that the transport time was resolved to 21±1 ms (62 events) for β-actin mRNPs and 16±2 ms (65 events) for firefly luciferase mRNPs ( Table 1 ). Second, capability of localizing a single NPC on the NE with high localization precision. SPEED microscopy only illuminates a single NPC embedded in the NE of living cells. The centroid position of the imaged single NPC is localized with 1–3 nm precision in permeabilized cells and 5–11 nm in living cells. By contrast, wide-field epi-fluorescence microscopy simultaneously excites multiple proximal GFP-NPCs on the NE ( Supplementary Fig. S6 ). The resulting, heavily overlapping diffraction-limited fluorescent spots of GFP-NPCs form a continuous fluorescent NE, complicating an accurate determination of the NE middle plane or the centroid of individual NPCs on the NE ( Supplementary Fig. S6 ). In addition, many slowly moving or even immobile mRNPs reside around the periphery of the NE on either the nuclear or cytoplasmic side ( Table 2 , Supplementary Fig. S7 and Supplementary Movie 3 ). With a less accurately determined NE middle plane or NPC centroid, one would inevitably have difficulty to determine whether some mRNPs move inside or outside an NPC, and thus one may include some mRNPs that do not undergo export through the NPC. To further explore the above problems, we measured the dwell times of mRNPs outside the NPC, including mRNPs that interacted with NPC-deficient regions on the NE, or moved within the nucleus or cytoplasm. Their dwell times were determined to be as long as hundreds of milliseconds or even seconds ( Table 1 and Supplementary Movie 3 ). Two-dimensional maps of nuclear mRNP export through the NPC Altogether, 2,379 spatial localizations from export events of firefly luciferase mRNPs through 20 NPCs from 20 cells were superimposed to obtain the two-dimensional (2D) spatial distribution map of Fig. 2a , which identified a void space at the position of the NE, as expected. The binned histogram of mRNP locations along the NPC axis indicated more localizations on both the nucleoplasmic (−120 to −20 nm) and cytoplasmic sides (20–120 nm) compared with the NPC centre (−20 to 20 nm), a distribution that could be fitted with two Gaussian functions ( Fig. 2b ). These concentrated localizations of mRNPs on either side of the NPC were previously observed and assigned to cofactor assembly and disassembly processes, respectively [3] . However, we observed similarly clustered localizations for passively diffusing GFP and a Tap ΔNLS –p15 complex (here the transport receptor Tap lacks an nuclear localization signal (NLS) to prevent complex formation with NLS-related transport receptors, such as Importins α and β1 (ref. 30 ), neither of which requires such (dis)assembly ( Fig. 2d–h ). Given the diffusion volumes of these transiting substrates in each sub-region of an NPC gained from their cumulative 3D transport paths through the NPC ( Fig. 3 ), their highest spatial density appears at the geometric narrowest centre, instead of both ends, of the NPC ( Fig. 2c,f,i ). We therefore conclude that assembly and disassembly of mRNPs unlikely cause the two localization clusters observed here. Rather, they are simply results from the geometric constraints imposed by the NPC that allows for more spatial dwellings outside its narrow centre [27] , [28] . Figure 2: 2D spatial distribution of molecular locations in the NPC. ( a ) Experimentally determined 2D spatial locations of mRNPs in the NPC. A schematic of the NPC (light blue) is superimposed, and the central region of the NPC (−20 nm to 20 nm) is highlighted in yellow. C, cytoplasmic side of the NPC; N, nucleoplasmic side of the NPC. ( b ) Gaussian fitting of the binned histogram of spatial mRNP locations along the NPC axis ( x dimension) produced two major peaks on either side of the NPC. Approximately 13% of total localizations fall in the central channel of the NPC (−20 to 20 nm). ( c ) Density of spatial locations along x dimension. ( d – f ) The 2D spatial locations, binned histogram of spatial locations along the NPC axis and corresponding spatial density for Tap ΔNLS –p15. ( g – i ) The 2D spatial locations, binned histogram of spatial locations along the NPC axis and corresponding spatial density for GFP. 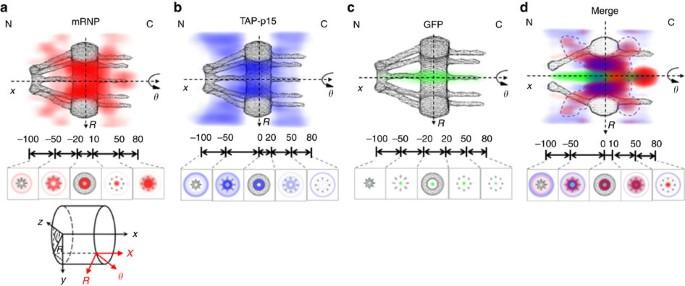Figure 3: 3D spatial probability density maps. (a) 3D spatial density map of mRNPs (red, deeper shade indicates higher density), generated using a 2D-to-3D deconvolution algorithm, is shown in both a cut-away and a cross-section view superimposed on the NPC architecture (grey). Five regions with distinct spatial location distributions for mRNPs are marked with relative distances (in nm) from the centroid of the NPC. Cartesian (x,y,z) and cylindrical (x,R,θ) coordinate systems are shown. C, cytoplasmic side of the NPC; N, nucleoplasmic side of the NPC. (b) Cut-away and cross-section views of the 3D spatial density map for the TapΔNLS–p15 heterodimer (blue, deeper shade indicates higher density) superimposed on the NPC architecture (grey). (c) Cut-away and cross-section views of the 3D spatial density map for passively diffusing GFP molecules (green, deeper shade indicates higher density) superimposed on the NPC architecture (grey). (d) Merged maps of the three transport routes through the NPC. The regions overlapping between mRNP and TapΔNLS–p15 are outlined with dashed lines. Full size image Figure 3: 3D spatial probability density maps. ( a ) 3D spatial density map of mRNPs (red, deeper shade indicates higher density), generated using a 2D-to-3D deconvolution algorithm, is shown in both a cut-away and a cross-section view superimposed on the NPC architecture (grey). Five regions with distinct spatial location distributions for mRNPs are marked with relative distances (in nm) from the centroid of the NPC. Cartesian ( x , y , z ) and cylindrical ( x , R , θ ) coordinate systems are shown. C, cytoplasmic side of the NPC; N, nucleoplasmic side of the NPC. ( b ) Cut-away and cross-section views of the 3D spatial density map for the Tap ΔNLS –p15 heterodimer (blue, deeper shade indicates higher density) superimposed on the NPC architecture (grey). ( c ) Cut-away and cross-section views of the 3D spatial density map for passively diffusing GFP molecules (green, deeper shade indicates higher density) superimposed on the NPC architecture (grey). ( d ) Merged maps of the three transport routes through the NPC. The regions overlapping between mRNP and Tap ΔNLS –p15 are outlined with dashed lines. Full size image Diffusion patterns of mRNPs inside and outside the NPC To gain further insight into the diffusive behaviour of mRNPs in living cells, we determined the diffusion coefficients of mRNPs inside and outside the NPC. First, hundreds of single-molecule trajectories for individual mRNPs in either the cytoplasm or nucleus were captured with a detection speed of 500 frames per second. The obtained mean squared displacements (MSDs) of mRNPs revealed that nuclear mRNPs possess multiple diffusion coefficients of 3.42 μm 2 s −1 (23%) and 0.61 μm 2 s −1 (67%), and nearly stationary coefficients of 0.09 μm 2 s −1 (7%) and 0.03 μm 2 s −1 (3%); cytoplasmic mRNPs diffuse at 2.24 μm 2 s −1 (57%), 0.34 μm 2 s −1 (38%) and 0.05 μm 2 s −1 (5%). As shown in Table 2 , the diffusion coefficients that we obtained for slowly moving or immobile mRNP events agree well with previous reports [3] , [6] , [7] , [31] , [32] . However, our measurements discovered that a significant fraction of mRNPs conducts much faster diffusion in both cytoplasm and nucleus that escaped previous detection at lower speeds. For confirmation, we adopted a 50-fold slower detection speed (100 ms per frame) to repeat the diffusion measurements for mRNPs in both cellular compartments. As expected, only more slowly diffusing mRNPs were observed ( Supplementary Fig. S3 and Table 2 ). The multiple diffusion coefficients observed for mRNPs in both cytoplasm and nucleus suggest that mRNPs diffuse through highly heterogeneous microenvironments formed in these cellular compartments, where some particles remain stationary, whereas others adopt diffusion patterns as diverse as corralled, Brownian and biased diffusion ( Supplementary Fig. S3 and Table 2 ). In contrast to our measurements in the nucleus and cytoplasm, the determination of mRNP diffusion constants in the sub-micrometre-sized NPC is complicated by the geometric constraints of the NPC and the short nuclear export time. To better evaluate the diffusive patterns of mRNPs, we experimentally determined their diffusion coefficients in each sub-region of the NPC. Given the 12-ms total nuclear export time of mRNPs ( Fig. 1 ) and the ratio between the spatial locations in sub-regions of the NPC ( Fig. 2 ), we estimated the dwell times of mRNPs in each sub-region of the NPC to be ~5.5 ms on the nucleoplasmic side, ~1.6 ms in the central region and ~4.9 ms on the cytoplasmic side (Methods). With the diffusion volumes of mRNPs in each sub-region of an NPC obtained from their cumulative 3D transport routes through the NPC ( Fig. 3 ), we determined the diffusion constants of mRNPs exporting through the NPC to ~0.16 μm 2 s −1 on the nucleocytoplasmic side, ~0.07 μm 2 s −1 while crossing the pore centre and ~0.19 μm 2 s −1 on the cytoplasmic side of the NPC (Methods). Clearly, these results suggest that mRNPs diffuse faster on both sides but slower through the centre of the NPC, opposite to a previous proposal based on intracellular single-particle tracking [6] , but consistent with the previous suggestion of a physical/entropy barrier in the crowded NPC centre [33] , [34] . 3D transport routes of mRNPs through the NPC Our recent studies have shown that the determination of the nucleocytoplasmic transport pathways based solely on 1D or 2D spatial localizations is incomplete [27] , [28] , [29] . Following well-established deconvolution procedures exploiting the cylindrical symmetry of the NPC [27] , [28] , [29] , we therefore converted our 2D spatial distributions of mRNPs, Tap ΔNLS –p15 and GFP in the NPC ( Fig. 2a ) into their corresponding 3D probability density maps ( Fig. 3 and Supplementary Movies 4–7 ). Comparison of the 3D maps revealed that mRNPs translocate through the periphery around a rarely entered central axial channel of the NPC before they dissociate on the cytoplasmic side. Strikingly, mRNPs and Tap ΔNLS –p15 show major overlap between their export pathways, particularly in the NPC centre and on the nucleoplasmic side ( Fig. 3d ), consistent with the fact that Tap–p15 mediates the interaction of mRNPs with the FG Nups on the nucleoplasmic face and in the central region of the NPC [2] . The diameter of the unoccupied channel at the cross-section of the NPC centre is 10±1 nm for mRNPs and 15±1 nm for Tap–p15, indicating that the larger mRNPs still do not occupy the entire volume of the NPC. By contrast, this central axial channel is utilized by the passively diffusing GFP ( Fig. 3c ). In agreement with previous conclusions [27] , passively diffusing molecules such as GFP (or mCherry) take a path consistent with size confinement in the central channel of the NPC [35] , whereas mRNPs and Tap–p15 conquer the central dense FG-repeat barrier anchored at the central channel wall. Both types of interaction, however, lead to the observed decelerated diffusion through the NPC centre. After passing through the central NPC region, mRNPs start to broadly diffuse around the cytoplasmic fibrils and invade the passive diffusion channel on the cytoplasmic side ( Fig. 3a ), differing thus from the Tap ΔNLS –p15 paths. This difference is consistent with the previous proposal that DDX and other transport cofactors like Dbp5 and Gle1 disassemble the mRNP:Tap–p15 complex from Nup214 on the cytoplasmic side of the NPC [36] , [37] , a process that may not be required for Tap–p15 alone. We propose that mRNPs dissociate from the NPC in this zone, 50–80 nm into the cytoplasmic side. These mRNP transport routes provide the first real-time 3D view of such a large and complex cargo exported through the NPC in living cells under the native conditions of intrinsically disordered FG Nups, which are inevitably distorted or damaged in frozen or chemically fixed cells [38] . To ask what impact Tap–p15 association has on the export efficiency of mRNPs, we determined the export efficiency of Tap ΔNLS –p15 alone to be ~50%, consistent with the transport efficiencies of other receptors such as Crm1 and Importin β1 ( Supplementary Table S1 ) [27] , [28] . Moreover, the NPC acquiesces only ~50% transport efficiency for either passively diffusing molecules, such as GFP, or Importin β1-facilitated translocation of cargo complex ( Supplementary Table S1 ) [27] , [28] , [39] . That is, only half of all incoming molecules successfully pass through the NPC under normal physiological conditions during both passive and facilitated transport. Although the process of transport in living cells may be more complex than that in permeabilized cells, previous studies have shown similar nucleocytoplasmic transport times and efficiencies for either cargo-bound or cargo-free transport receptors when comparing permeabilized and living HeLa cells [39] , [40] . We therefore propose that only an additional ~14%, rather than ~64%, of all mRNP export attempts (corresponding to ~22% of all abortive events) are rejected by the NPC’s central channel. The lower abortive probability and shorter export time determined here suggest a more efficient mRNP nuclear export in living cells than previously thought. Together with the recently reported nuclear membrane budding [9] , our findings have important consequences for our understanding of how efficiently genetic information can flow in eukaryotic cells to support their viability and growth. Location of the mRNP selectivity barrier Finally, to understand the mechanism of mRNP selectivity, we compared the spatial distributions of successful and abortive mRNP export events ( Fig. 4 ). The superimposed trajectories of 38 successful mRNP export events showed a peak centred around 47 nm into the cytoplasmic side. The deepest penetrations of these events inevitably move beyond the central region (−20 to 20 nm) and reach the cytoplamic side of the NPC (20–120 nm). By contrast, the spatial locations of 50 abortive export events form a peak around −115 nm on the nuclear side. In addition, the localizations of 80% of these mRNPs are restricted to the nuclear side and the central region (−120 to 20 nm). These results suggest that mRNPs only gain a high probabilty to complete their nuclear export once they transverse the NPC centre. Notably, recent studies have shown that protein cargo molecules larger than the cut-off size of passive diffusion (>40–60 kDa) are similarly restricted by the NPC central region [20] , [27] , [28] , suggesting that this region generally serves as the critical selection barrier for all actively translocated cargo molecules. Previous studies have shown that both the assembly of mRNPs at the nuclear basket and the dissociation of the mRNP complex on the cytoplasmic side have important roles in the quality control of nuclear export [1] , [2] , [3] , [4] , [5] , [41] . Here we revealed that the central pore region of the NPC serves as another critical control for mRNP export. Together, these three steps may function as a sequential series of quality-control processes rate-limiting nuclear mRNP export. 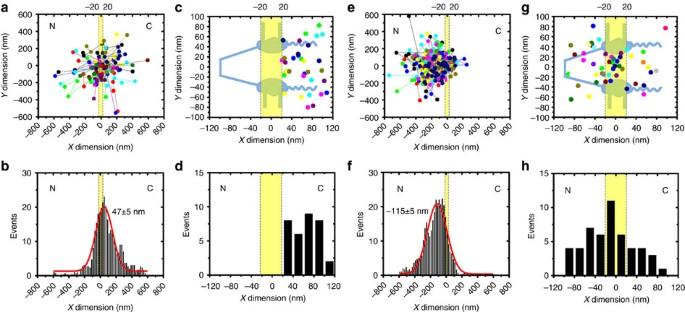Figure 4: Single-molecule trajectories of successful and abortive mRNP export events. (a) Superimposed single-molecule trajectories of 38 successful mRNP export events. The central region of the NPC (−20 to 20 nm) is highlighted in yellow. C, cytoplasm; N, nucleoplasm. (b) The binned histogram of spatial locations for the successful mRNP export events along the NPC axis was fitted by a Gaussian function to yield a peak at position 47±5 nm on the cytoplasmic side. (c) Spatial locations of the last stage of the successful mRNP export events shown ina. (d) Binned histogram of locations inc. (e) Superimposed single-molecule trajectories of 50 abortive mRNP export events. (f) The binned histogram of spatial locations for the abortive mRNP export events inewas fitted by a Gaussian function to yield a peak at position −115±5 nm on the nucleoplasmic side. (g) Spatial locations of the deepest penetration steps for the abortive mRNP export events shown ine. (h) Binned histogram of locations ing. Figure 4: Single-molecule trajectories of successful and abortive mRNP export events. ( a ) Superimposed single-molecule trajectories of 38 successful mRNP export events. The central region of the NPC (−20 to 20 nm) is highlighted in yellow. C, cytoplasm; N, nucleoplasm. ( b ) The binned histogram of spatial locations for the successful mRNP export events along the NPC axis was fitted by a Gaussian function to yield a peak at position 47±5 nm on the cytoplasmic side. ( c ) Spatial locations of the last stage of the successful mRNP export events shown in a . ( d ) Binned histogram of locations in c . ( e ) Superimposed single-molecule trajectories of 50 abortive mRNP export events. ( f ) The binned histogram of spatial locations for the abortive mRNP export events in e was fitted by a Gaussian function to yield a peak at position −115±5 nm on the nucleoplasmic side. ( g ) Spatial locations of the deepest penetration steps for the abortive mRNP export events shown in e . ( h ) Binned histogram of locations in g . Full size image Exploiting the enhanced spatiotemporal super accuracy afforded by SPEED microscopy, we here have characterized the kinetics, 3D routes and selectivity mechanism for the export of mRNPs through the NPC. First, we have demonstrated that the central FG Nups of the NPC function as the major selective barrier for nuclear export of mRNPs. Only about 36% of all mRNPs entering the NPC from the nucleus successfully complete their export after accessing this central selective barrier, whereas the remaining mRNPs abort their export after interacting with the FG filaments in the central and nucleoplasmic regions of the NPC. Accordingly, we found that mRNPs adopt a fast-slow-fast diffusion pattern through the NPC, moving faster on either end and slower in the central region of the NPC, in direct opposition to the previous proposal that mRNP diffusion is attenuated in both peripheral regions of the NPC, but not its centre [3] , [6] . Second, mRNPs only need ~12 ms for transit through the NPC, 10 times shorter than previously suggested [6] . This much faster nuclear export was observed for both firefly luciferase and β-actin mRNP in living cells ( Table 1 ), the latter chosen for direct comparison with the previous work that found ~10-fold slower export times for this mRNA/cell line combination [6] . Third, reconstructions of the 3D export routes in living cells revealed that large mRNP complexes primarily interact with the periphery of the nucleoplasmic side and the centre of the NPC, only rarely occupying the central axial channel utilized for passive diffusion, and eventually dissociate on the cytoplasmic side. The latter results invoke a multilane traffic model wherein the signal-independent passive diffusion of small molecules and the transport receptor facilitated diffusion of large mRNP complexes follow distinct transport paths through the NPC [27] , [28] , [29] , [42] , [43] . SPEED microscopy has thus proven to be a powerful tool to study nucleocytoplasmic transport of proteins and mRNPs in vitro and in vivo [27] , [28] , [29] . In the future, the method can be expanded to other types and/or sizes of RNPs, or to the observation of conformational changes associated with their transport though the NPC. Cell culture and transport conditions Our genetically engineered HeLa cell line expresses stably GFP-conjugated POM121 and transiently mCherry-tagged firefly luciferase mRNA. More specifically, POM121, a structural Nup anchored at the central scaffold of the NPC, was genetically fused to GFP. Firefly Luciferase mRNA was extended by 24 MS2 stem loops on the 3′ end, and each loop was the binding target of an MS2-coating protein (MCP) dimer fused to mCherry. pMCP-EGFP, a plasmid bearing the open reading frame (ORF) of the MCP fused to EGFP and an SV-40 NLS, and pSL-MS2_24 × , a plasmid bearing 24 copies of the MS2 stem loops, were received as generous gifts from Robert Singer (Albert Einstein College of Medicine). The GFP ORF in pMCP-GFP was replaced with PCR-amplified mCherry ORF bearing Age I and Bsr GI restriction enzyme sites, to result in pMCP-mCherry. A Luciferase reporter plasmid bearing the MS2 stem loops was created in two steps. First, the ORF of IF2, PCR-amplified using a forward primer bearing Sbf I and Eco RI restriction enzyme sites and a reverse primer bearing a Not I restriction enzyme site, was cloned into the corresponding Sbf I and Not I sites in plasmid pmiR-GLO (Promega). Twenty-four copies of the MS2 stem loop from pSL-MS2_24 × were then cloned into the Eco RI– Not I restriction enzyme sites of the resultant plasmid, pmG-IF2, to generate pmG-MS2. Clones containing the MS2 stem loops were created in SURE2 bacterial cells (Stratagene) to minimize recombination of the MS2 repeats with the bacterial genome. Still, we had to resort to a two-step cloning procedure, as linearized plasmids containing the MS2 stem loops often recombined with the genome of competent bacterial cells, thus resulting in clones bearing smaller plasmids. The NLS was added to MCP to promote its import into the nucleus and enhance sufficient labelling of mRNAs even at the desired low MCP expression level. Freshly split HeLa cells were grown overnight on coverslips in DMEM (Grand Island, NY) supplemented with 10 mg ml −1 streptomycin, 100 U ml −1 penicillin and 10% newborn calf serum, at 37 °C, in a 5% CO 2 incubator. Extensive control experiments showed that eight copies of POM121 in the selected NPCs were labelled with GFPs ( Supplementary Fig. S1 ), and each mRNP complex imaged in our experiments was tagged with ~10 GFP or mCherry molecules ( Supplementary Fig. S2 ; this number of fluorescent protein molecules per mRNP was also expected because of using a tagging procedure similar to the one pioneered by Singer). Sequences of fluorescence images of GFP and mCherry were used to localize the centroid of the NPC and track mRNP export in living cells, respectively. Single-molecule imaging and tracking experiments of the nuclear export of labelled mRNPs were conducted in living cells, whereas the nucleocytoplasmic transport of Alexa Fluor 647-labelled Tap–p15 and GFP was imaged in digitonin-permeabilized cells. For the experiments conducted in permeabilized cells, flow chambers were constructed with a top coverslip and two lines of silicone grease as spacers. Cells were washed with transport buffer (20 mM HEPES-KOH, 110 mM KOAc, 5 mM NaOAc, 2 mM Mg(OAc) 2 and 1 mM EGTA (pH 7.3)), permeabilized for 2 min with 40 μg ml −1 digitonin in transport buffer and washed again with transport buffer supplemented with 1.5% polyvinylpyrrolidone (360 kDa). Polyvinylpyrrolidone was included in all transport buffer solutions after digitonin treatment to prevent osmotic swelling of nuclei. SPEED microscopy The SPEED microscope consists of an Olympus IX81 equipped with a 1.4 numerical aperture × 100 oil-immersion apochromatic objective (UPLSAPO 100XO; Olympus), a 35-mW 633-nm HeNe laser (Melles Griot), an on-chip multiplication gain CCD camera (Cascade 128 + ; Roper Scientific), two 120 mW ArKr tunable ion lasers (Melles Griot) and the Slidebook software package (Intelligent Imaging Innovations) for data acquisition and processing. An optical chopper (Newport) was used to generate an on–off mode of laser excitation. GFP, YFP, mCherry, tdTomato and Alexa Fluor 647 were excited by 488, 568 and 633 nm lasers, respectively. To minimize alignment problems in dual-colour measurements, both green and red fluorescence emissions were collected by the same objective, filtered by a dichroic filter (Di01-R405/488/561/635-25 × 36; Semrock) and an emission filter (NF01-405/488/561/635-25 × 5.0; Semrock), and imaged by an identical Cascade 128 + CCD camera successively. Proteins and labelling GFP and human Tap ΔNLS –p15 heterodimer proteins were expressed in Escherichia coli and purified by Ni-NTA Superflow (Qiagen), MonoQ and Superdex 200 (Amersham) chromatography. The solvent accessible cysteines on the proteins were labelled with a 20-fold molar excess of Alexa647 maleimide dye (Invitrogen) for 2 h at room temperature in 50 mM sodium phosphate and 150 mM NaCl (pH 7.5). Reactions were quenched with 2-mercaptoethanol, and the products were dialyzed to remove the free dye. The labelling ratio was about two dye molecules per TapΔNLS/p15 heterodimer, and one dye per GFP. Copy number of MCP-FPs per mRNP and mRNP size To determine the copy number of MCP-FP molecules per mRNP, we quantified the fluorescence of a GFP and that of NPCs with eight copies of GFP-POM121 in vitro , and GFP-MCP-mRNP in vivo , each at the single-molecule level. As shown in Supplementary Fig. S2 , each mRNP detected in our cell system has 9–10 copies of GFP-MCP, which agrees well with previous reports in a similar MS2-mRNP cell system [6] . The mRNA with the 24 MS2 loops has a length of ~3.3 kb (about 1.5 MDa), and each attached GFP-MCP is 39 kDa. With multiple endogenous proteins bound to the mRNA, the final average mass of the mRNPs is estimated to be 4–5 MDa, with a corresponding diameter of up to ~25 nm when assuming a roughly spherical shape. Determination of diffusion coefficients outside the NPC All videos were deconvolved using a 2D blind deconvolution routine in AutoQuantX3. Single particles were tracked as described [44] . Briefly, Imaris (Bitplane) was used for particle tracking. Only particles that lasted for more than nine frames were used for further analysis. All tracks were visually inspected to ensure that they arose from well-isolated particles. In-house MATLAB routines were used to calculate the MSD and diffusion coefficients. Brownian diffusion coefficients were calculated by fitting the MSD for the first three time intervals to the equation [45] : where represents the MSD, D represents the diffusion coefficient and Δ t represents time intervals. The MSD versus time plots were fitted using equations representing the appropriate diffusive motion as described [44] ( Supplementary Fig. S3 ). Transport times and diffusion coefficients of mRNPs inside the NPC Experimentally, mRNPs exhibited ~13% of their total spatial locations in the NPC centre, ~46% on the nucleoplasmic side and ~41% on the cytoplasmic side during the total ~12 ms transport time. Correspondingly, they spent ~1.6 ms in the centre, ~5.5 ms on nuclear side and ~4.9 ms on cytoplasmic side. The volume ( V ) in the NPC centre ( r cen , 25 nm in radius; L cen , 40 nm in length) is ~20 times smaller than that on either side of the NPC ( r cyto = r nuc , 80 nm in radius; L cyto = L nuc , 80 nm in length). The volume of a central channel ( r h , 10 nm in radius) barely occupied by mRNPs on the nucleoplasmic side and at the central region was subtracted from the calculation of diffusion volumes in these two areas. According to the following equations: the diffusion constants of mRNPs on the nucleoplasmic side, the centre and the cytoplasmic side of the NPC are D nuc =0.16 μm 2 s −1 , D cen =0.07 μm 2 s −1 and D cyto =0.19 μm 2 s −1 . Localization of the NE and NPC orientation The position of the NE was determined at super accuracy by fitting the fluorescence of GFP-POM121 as follows. The pixel intensities within a row or a column approximately perpendicular to the NE were fit with a Gaussian. The peak position of the Gaussian for a particular set of pixel intensities was considered the NE position for that row and column. The peak positions of a series of such Gaussians were then fit with a second-degree polynomial, yielding the orientation of the NE within the entire image. The following rules were then used to select a single NPC and determine its orientation, which needs to be perpendicular to the NE on the equator of the nucleus and to the y direction of the Cartesian coordinates ( x , y ) in the CCD camera: first, to focus on a GFP-NPC with eight copies of GFP-POM121, individual GFP-NPCs on the NE were selected when their fluorescence intensity was ~8-fold that of a single GFP; second, we chose a fluorescent NPC on the equator of the nucleus such that the tangent of the NE at the location of this NPC was parallel to the y direction of the Cartesian coordinates ( x , y ) in the CCD camera; and third, we examined the ratio of Gaussian widths in the long and short axes of the chosen GFP-NPC fluorescence spot, which needed to fall between 1.74 and 1.82. Within this range, an illuminated NPC only has a free angle of 1.4° to the perpendicular direction to the NE [28] . Localization precision of isolated fluorescent spots The localization precision for fluorescent NPCs, as well as immobile and moving fluorescent mRNPs, was defined as how precisely the central point of each detected fluorescent diffraction-limited spot was determined. For fluorescent NPCs and immobile mRNPs, the fluorescent spot was fitted with a 2D elliptical and symmetrical Gaussian, respectively, and the localization precision was determined by the s.d. of multiple measurements of the central point. For moving mRNPs, the fluorescent spot was fitted with a 2D elliptical Gaussian function, and the localization precision ( σ ) was determined as: , where N is the number of collected photons, a is the effective pixel size of the detector, b is the s.d. of the background in photons per pixel and s is the s.d. of the point spread function [46] . To verify the precision as obtained from the s.d. of multiple measurements and the above equation, both methods were used to determine the localizations of immobile fluorescent molecules (Alexa Fluor 647-labelled-GFP absorbed on the surface of a coverslip) and fluorescent NPCs. A total of 230 immobile GFP-labelled molecules were measured, and the two methods yielded a difference of 0.5±0.1 nm. In our measurements, typically 3,000 signal photons versus 15 noise photons were collected from individual 10-mCherry-labelled mRNPs at a detection frame rate of 500 Hz in living cells. Correspondingly, the localization precision was ~8 nm for the immobile single mRNPs and ~10 nm for moving mRNPs. Because of the inevitable vibration of NPCs in the NE of living cells, the localization precision of the NPC centroid was 5–11 nm. In addition, based on the detection of 230 immobile Alexa647-labelled GFP molecules adsorbed on a coverslip, the system error of aligned red and green fluorescence channels was determined to be 3.0±0.1 nm. Therefore, the overall tracking precision for mCherry-fused mRNP export through the GFP-labelled NPC in living cells was estimated to be ~11–15 nm. Deconvolution and 3D image processing The detailed deconvolution process used to obtain the 3D spatial probability density maps of particles transiting through the NPC was described in our previous publications [20] , [27] , [28] , [29] . In short, the 3D spatial locations of molecules transiting through the NPC can be considered in either Cartesian ( x , y , z ) or cylindrical ( x , r , θ ) coordinates. In microscopic imaging, the observed 2D spatial distribution of particle localizations is a projection of its actual 3D spatial locations onto the x–y plane. The underlying 3D spatial distributions can be recovered by projection of the measured Cartesian ( x , y ) coordinates back onto the simplified cylindrical ( r , x ) coordinates, based on the expected cylindrically symmetric distribution along the θ direction of the nuclear pore [28] . The resulting 3D, surface-rendered visualizations shown in figures and movies were generated with Amira 5.2 (Visage Imaging). Statistics Experimental measurements are reported as mean±s.e.m., unless otherwise noted. How to cite this article: Ma, J. et al . High-resolution three-dimensional mapping of mRNA export through the nuclear pore. Nat. Commun. 4:2414 doi: 10.1038/ncomms3414 (2013).